High-density waveguide superlattices with low crosstalk Silicon photonics holds great promise for low-cost large-scale photonic integration. In its future development, integration density will play an ever-increasing role in a way similar to that witnessed in integrated circuits. Waveguides are perhaps the most ubiquitous component in silicon photonics. As such, the density of waveguide elements is expected to have a crucial influence on the integration density of a silicon photonic chip. A solution to high-density waveguide integration with minimal impact on other performance metrics such as crosstalk remains a vital issue in many applications. Here, we propose a waveguide superlattice and demonstrate advanced superlattice design concepts such as interlacing-recombination that enable high-density waveguide integration at a half-wavelength pitch with low crosstalk. Such waveguide superlattices can potentially lead to significant reduction in on-chip estate for waveguide elements and salient enhancement of performance for important applications, opening up possibilities for half-wavelength-pitch optical-phased arrays and ultra-dense space-division multiplexing. Silicon photonics has made great strides in developing a wide range of devices [1] , [2] , [3] , [4] , [5] , [6] , [7] , [8] , [9] , [10] , [11] , [12] , [13] . Built upon these advances, this technology now offers a low-cost platform for building large-scale optical systems [14] , [15] , [16] , [17] . Waveguide arrays are among the cornerstones of such systems. For example, waveguide arrays are widely used in emerging applications such as optical-phased arrays [18] , [19] , [20] , [21] , space-division multiplexing [22] and chip-scale optical interconnects [23] , [24] , and conventional applications such as wavelength-division multiplexers [25] , [26] . On the other hand, a waveguide array or a waveguide lattice can also be viewed [27] as fully analogous to a periodic chain of atoms, which lends itself to a broad spectrum of fascinating scientific possibilities ranging from Anderson localization of light [28] , [29] to parity-time symmetric effects [30] . Thus far, in most studies, the pitch associated with such relatively simple waveguide arrays/lattices has been typically large, ranging from a few micrometres to tens of micrometres (or a multiple of wavelengths) [18] , [19] , [21] , [31] , [32] . As such, the inter-coupling between waveguides can be generally weak, which helps to reduce crosstalk. On the other hand, the subwavelength- or submicron-pitch regime of such systems has not been adequately explored for practical applications, mainly because of an intolerable surge in crosstalk usually occurring at these length scales. Here we introduce a superlattice of waveguides, whose supercell comprises a sub-array of waveguides, and explore intricate light inter-coupling and scattering in such a system. Guided by physical insight and advanced simulations, we introduce a set of superlattice design principles dedicated to crosstalk reduction. Especially, through an interlacing-recombination supercell design scheme, we demonstrate the possibility for very weak crosstalk even as the waveguide pitch reaches the half-wavelength scale. This not only enables high-density integration of waveguide elements with potential significant reduction in on-chip estate and cost, but also helps to improve the performance for important devices such as finer wavelength resolution for wavelength de-multiplexers. Furthermore, high-density waveguide superlattices may open up opportunities for half-wavelength-pitch optical-phased arrays and ultra-dense space-division multiplexing that have long been sought. Crosstalk from coupling beyond nearest neighbours The smallest possible waveguide array is a pair of waveguides. Low crosstalk can be easily achieved for such a pair at small spacing on the basis of the asymmetric directional coupler theory. In such a coupler, it is well known that the normalized power coupling (that is, crosstalk) from one waveguide to another is given by ref. 33 , where Δ β represents the propagation constant difference (or phase mismatch) between two waveguides, κ the coupling strength and L the propagation distance. The maximum crosstalk is given by ( ). One readily sees that if the phase mismatch is large (Δ β >> κ ), the crosstalk can be low. Although the above theory has been known for a long time, there is no clear route to scale it up to offer a crosstalk solution for a large array. Note that scalability is a key factor for any technology advance in integrated electronics/photonics: a technology that can be used in large-scale integration is much more valuable than one applicable only on small scale [34] . Crosstalk in a large array of waveguides is fundamentally different because light in one waveguide of the array can be transported to the second-, third-nearest waveguide-neighbours and beyond (particularly, at sub-λ pitches, the mode overlap with second-, third-nearest waveguide-neighbours is not negligible and crosstalk will rise). Such transport can comprise contributions from multiple indirect coupling paths (for example, between waveguides #1 and #4, light can be coupled from waveguide #1 to #2 then to #4, or from #1 to #3 then to #4). Crosstalk due to a superposition of all these coupling paths cannot be deterred by any known approach. However, when an artificial periodic structure is introduced into a waveguide array to form a superlattice as shown in Fig. 1 , a hierarchy of crosstalk at intra-supercell and inter-supercell levels is formed. As such, the crosstalk treatment can be divided into two levels: first find an optimal design to minimize crosstalk in each supercell, which has a limited number of coupling paths; then consider inter-supercell crosstalk, which is generally much weaker for sufficiently large supercells. Note that it is easy to verify that superlattices based on small, trivial supercells (for example, containing two waveguides) still have strong crosstalk at sub-micrometre pitches (see examples in Supplementary Fig. 1 ). Hence, it is necessary to explore large, sophisticated supercell structures. 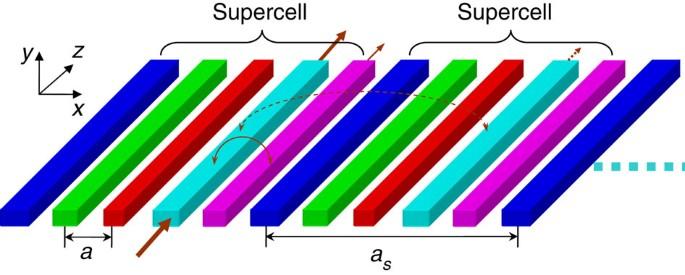Figure 1: Schematic drawing of a waveguide superlattice.  Figure 1: Schematic drawing of a waveguide superlattice. Full size image Physics and design principles of low-crosstalk superlattices To explore sophisticated superlattice structures for crosstalk suppression, we need to first understand the physics of light transport in such a superlattice so as to develop rational design principles as well as accurate theoretical tools for crosstalk simulation. First, to build a superlattice, we need different species of ‘atoms.’ Here, we choose waveguides of different widths w because such ‘atoms’ can be fabricated relatively easily by the VLSI technology. More types of such ‘atoms’ are clearly desirable for creating more sophisticated superlattice designs. However, there are two physical constraints that limit the range of available waveguide widths. On one hand, the maximum waveguide width is constrained by the single-mode condition ( w max ∼ 450 nm here). On the other hand, for a very narrow waveguide, the width of the optical mode increases significantly as the waveguide width decreases. This, in turn, enlarges the mode overlap between neighbouring waveguides, and enhances their inter-coupling strength κ n,n + k ( k =±1, ±2,…). Eventually, at a sufficiently narrow w , crosstalk starts to increase because the increase in κ n,n+k cancels out any benefit introduced by increasing Δ β . This effect can be illustrated by a special case, a pair of waveguides, in which only the nearest-neighbour coupling is present. 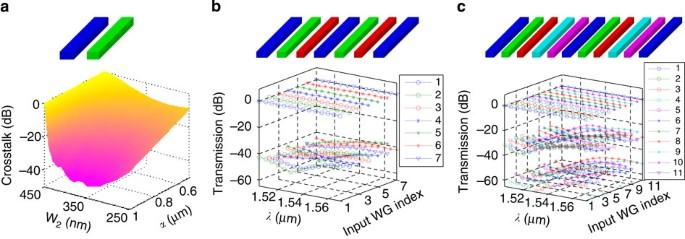Figure 2: Simulated crosstalk due to inter-coupling between waveguides. (a) Maximum crosstalk between a pair of waveguides of different widths (w1=450 nm,w2and pitchavary) atλ=1,550 nm. (b) SC3 superlattice,a=1 μm,L=200 μm. (c) SC5 superlattice,a=0.8 μm,L=200 μm. Inbandc, transmission spectraTi,j(λ) from a given input waveguide (WG)ito different output waveguides are plotted in thei-th plane (for example,T1,jall in the first plane). The colour/symbol for each output channeljis shown in the legend. Figure 2a shows numerically calculated maximum crosstalk ( ) for a pair in which the first waveguide has a width of w 1 =450 nm and the second waveguide width, w 2 , is varied. Clearly, at a sufficiently narrow w 2 , crosstalk starts to increase (for a given pitch). Considering this limit and also noting that narrow waveguides tend to have higher loss (see loss information in Methods), the narrowest waveguide used in the superlattices is set to be ∼ 330 nm wide. Figure 2: Simulated crosstalk due to inter-coupling between waveguides. ( a ) Maximum crosstalk between a pair of waveguides of different widths ( w 1 =450 nm, w 2 and pitch a vary) at λ =1,550 nm. ( b ) SC3 superlattice, a =1 μm, L =200 μm. ( c ) SC5 superlattice, a =0.8 μm, L =200 μm. In b and c , transmission spectra T i,j ( λ ) from a given input waveguide (WG) i to different output waveguides are plotted in the i -th plane (for example, T 1 ,j all in the first plane). The colour/symbol for each output channel j is shown in the legend. Full size image Second, in a sophisticated superlattice, many effects come up due to complex light transport/coupling. For example, the inter-coupling causes the effective propagation constant Λ of a superlattice mode to deviate from the intrinsic β of an isolated waveguide. Furthermore, light transport may also comprise contribution from inter-waveguide scattering due to structure imperfections (for example, waveguide sidewall roughness), which will be discussed later as a secondary effect. Hence, a rigorous theory is needed to model light transport in a superlattice. Note that approximate theories based on small index contrast cannot be applied to silicon waveguides. Here, a fully vectorial waveguide mode theory previously developed for a high-index-contrast photonic crystal waveguide [35] , [36] is used. It can be shown that the amplitude of the mode, c n ′, can be obtained from where β n is the propagation constant of the original mode of the n -th waveguide, B mn is related to the overlap integral between modes m and n and Δ A mn is the perturbation potential matrix element (see detailed derivation of equation (10) in the Supplementary Note 1 ). In addition, n super denotes the number of waveguides in a supercell, and the superlattice period is given by a s = n super a . To include contributions of all coupling paths, a full matrix Δ A is used rather than limiting to the nearest-neighbours only (that is, only Δ A n , n ±1 ). Third, despite the complexity of superlattice coupling, some heuristic guidelines can be developed to design the superlattices. For example, while the propagation constants of the superlattice modes (Λ n ) deviate from those of the original waveguide modes ( β n ), our simulations indicate that the crosstalk between waveguide # m and # n tends to be small if Λ m −Λ n is sufficiently large. It can be further shown (see derivation of equation (12) in Supplementary Note 1 ) that two superlattice modes can have sufficient phase mismatch Λ m −Λ n if where [ K ]=[ B ] −1 [Δ A ]+[ β ] and [ β ] is a diagonal matrix whose elements are β n . The sums in the inequality indicate that all coupling terms, rather than only the nearest-neighbour coupling, must be considered to minimize the crosstalk in a waveguide array in general. Generally, if the ratio between the two sides in equation (2) is >10, the phase mismatch of two superlattice modes is sufficient to obstruct their coupling via a superposition of all coupling paths; and the crosstalk tends to be low. Note that each coupling matrix element Δ A mn is not a simple function of waveguide widths w m and w n (see, for example, Fig. 2a where the crosstalk is not a simple monotonous function of w 2 even for just two waveguides). As such, the above inequality regarding K mn cannot be further expressed in terms of waveguide widths w n . However, given the widths w m and pitch a , computing the K matrix takes little time compared with solving the differential equations as in equation (1). Therefore, this inequality helps to quickly rule out some structures without numerically solving equation (1), which is important when searching a large design space for the superlattice structures. Alternatively, one may also use to obtain an upper bound of the crosstalk between input waveguide # q and output waveguide # m , where u m ( L ) is the output amplitude and [ Q ] can be obtained from eigenvalue decomposition of [ K ] (see derivation of equation (14) in Supplementary Note 1 ). On the basis of these analyses, we first designed a superlattice with three waveguides in each supercell (called ‘SC3’ hereafter). By spreading the waveguide widths sparsely between the upper and lower bounds set above, we choose the waveguide widths to be 450, 380 and 330 nm. Simulations showed that the SC3 superlattice can achieve <−30 dB crosstalk between nearest neighbours at 1 μm pitch, as depicted in Fig. 2b . Such a SC3 superlattice with a pitch of 1 μm and a length of L =200 μm was fabricated on a silicon-on-insulator chip (fabrication processes, waveguide structure details, measurement schemes and waveguide loss are described in Methods. The ma-N e-beam resist was used here). The measured transmission spectra are shown in Fig. 3a . As a starting point, only two superlattice periods (plus one extra #7 for a rough estimate of crosstalk over 2 a s ) were studied to save time in simulation, fabrication and measurement. For light input into a given waveguide i , output spectra of all seven waveguides T ij ( λ ), j =1, 2,…,7, were measured (7 × 7=49 spectra in total for different i ). For a visual comparison of crosstalk between different channels, the transmission spectra originating from one input waveguide are normalized with respect to the peak transmission of the corresponding direct through channel (for example, T 3 j ( λ ) all normalized by the peak of T 33 ( λ )) so that each direct through channel has its peak aligned at 0 dB. Note that by defining the maximum crosstalk from channel i to channel j as , the crosstalk value is not affected by the normalization scheme of T ij . To avoid a heavily cluttered presentation, for each input, only the two nearest neighbours ( T i , i ±1 ) plus the worst crosstalk channel are plotted in Fig. 3a . Evidently, the crosstalk was fairly low. For ease of visual comparison, the statistics (mean and standard deviation) of each transmission spectrum T ij ( λ ) is plotted in Fig. 3b . Note that the true crosstalk for many channels should be very small (for example, T 26 <−80 dB) and is below the noise floor of our measurement setup (see noise floor discussion in Methods). The values of these channels were measured and shown in Fig. 3b just for verifying that its crosstalk was low enough for most applications. The overall crosstalk level of the leading crosstalk channels in Fig. 3b was several dB higher than the theoretical results in Fig. 2b , but it was still within a reasonable range considering the noise floor of our measurement setup and the noise due to scattering from sidewall roughness, which will be discussed later. The peaks of all crosstalk channels were in the range of −24 dB to −20 dB. However, when the pitch a is reduced below 1 μm, this SC3 structure produces significantly higher crosstalk. For example, for a SC3 superlattice with a =0.8 μm that we fabricated, the peak crosstalk channel XT max (2,5) can surge above −10 dB. 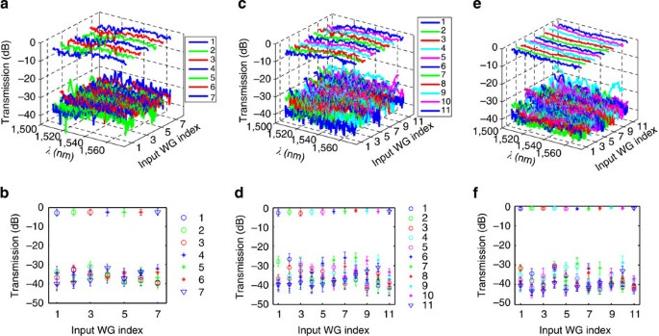Figure 3: Measured transmission spectra and their statistics for waveguide superlattices. (a–b) SC3 superlattice made by ma-N resist (a=1 μm,L=200 μm); (c–d) SC5 superlattice made by ma-N resist (a=0.8 μm,L=200 μm); (e–f) SC5 superlattice made by HSQ (a=0.8 μm,L=500 μm). Only adjacent channelsTi,i±1plus the worst crosstalk channel are shown ina,cande. Different colours mark different output ports, whose indices are shown in the legends. The spectral statistics of all transmission channels are shown by error bars inb,dandf, respectively. The colour/symbol for each output channel is shown in the legend. Figure 3: Measured transmission spectra and their statistics for waveguide superlattices. ( a – b ) SC3 superlattice made by ma-N resist ( a =1 μm, L =200 μm); ( c – d ) SC5 superlattice made by ma-N resist ( a =0.8 μm, L =200 μm); ( e – f ) SC5 superlattice made by HSQ ( a =0.8 μm, L =500 μm). Only adjacent channels T i,i ±1 plus the worst crosstalk channel are shown in a , c and e . Different colours mark different output ports, whose indices are shown in the legends. The spectral statistics of all transmission channels are shown by error bars in b , d and f , respectively. The colour/symbol for each output channel is shown in the legend. Full size image Advanced superlattice design concepts for submicron pitch To further reduce crosstalk in the sub-micrometre-pitch regime, simple expansion of the supercell size (for example, to SC4) will encounter significant challenges and new design concepts must be introduced. In fact, due to the constraint of the waveguide width range discussed above, a trivial insertion of an extra waveguide in this width range into a supercell will likely reduce minimum Δ w in the superlattice and hence reduce the phase mismatch between certain waveguides (for example, inserting a w =420 nm waveguide into the SC3 supercell above to expand to a SC4 supercell reduces the minimum Δ w to 30 nm). Interestingly, for n super >3, lower superlattice-level symmetry unleashes enormous design freedom through permutation of the waveguides in a supercell (Note that for n super ≤3, after classifying all permutations that are equivalent by translation/inversion symmetry, there is essentially one unique order once the set of waveguide widths are decided.). Consider the case of n super =5, and assume five waveguide widths satisfy w a > w b > w c > w d > w e . In this case, a simple descending (or ascending) order of the waveguide widths ( w a w b w c w d w e ) in a supercell is not optimal for crosstalk reduction. We discover that an interlacing-recombination configuration significantly reduces the crosstalk. In this configuration, two interlacing sub-arrays ( w a w c w e ) and ( w b w d ) of the original descending-ordered array recombine head to tail into a supercell ( w a w c w e w b w d ). As such, any two waveguides that have the least width difference (for example, w c and w b ) are separated by at least 2 a rather than a . This larger separation significantly reduces the crosstalk between these two waveguides that have the least phase mismatch. This is illustrated in Fig. 2c , which shows the simulation results for a SC5 superlattice whose supercell comprises 200 μm long waveguides of widths 450, 390, 330, 420 and 360 nm at pitch a =0.8 μm. Such a SC5 superlatttice was fabricated. Its measured spectra are shown in Fig. 3c and its spectral statistics (all 121 spectra) in Fig. 3d . Compared with the statistics of the SC3 superlattice at a =1 μm in Fig. 3b , the overall crosstalk level rose, substantially spreading into the −30 to −20 dB range. The trend is consistent with the theoretical results in Fig. 2b,c . Note that the overall maximum crosstalk XT max (7,6)=−18.8 dB is substantially above the theoretical prediction. The high maximum channel crosstalk in Fig. 3c can be attributed, in part, to the random light scattering between different waveguide modes due to sidewall roughness. Roughness-induced scattering loss has been studied in single waveguides [37] , [38] . In a waveguide superlattice, scattering can cause crosstalk fluctuation or noise. Detailed simulations show that the crosstalk fluctuation can be much reduced (see Supplementary Fig. 3 and Supplementary Note 2 ) if the sidewall roughness can be reduced. In light of this, we used an ultrafine-resolution e-beam resist hydrogen silsesquioxane (HSQ), instead of the previous moderate-resolution ma-N resist, to fabricate a 500-μm long SC5 superlattice. The measured spectra are depicted in Fig. 3e and their statistics in Fig. 3f . Compared with the SC5 superlattice in Fig. 3c,d , the standard deviations of the direct transmission spectra T ii are substantially reduced. This signifies a reduction of scattering-induced spectral noise (despite a longer L ). The diminishing scattering also helps to suppress the overall maximum crosstalk of the entire superlattice to XT max (10,9)=−21.1 dB at λ ∼ 1,565 nm. For reference, in a L =500 μm SC5 superlattice fabricated by the ma-N resist, the peak crosstalk of some channels rose above −15 dB. To further demonstrate the characteristics of the waveguide superlattice beyond two supercells, we have fabricated a 500-μm long superlattice of five SC5 supercells at a pitch of a =0.78 μm using HSQ e-beam resist. The transmission from each of the five waveguides in the centre supercell to its neighbouring 11 waveguides within one superlattice period was measured and plotted in Fig. 4 (for example, for input waveguide #12, output spectra from #7 to #17 were measured). Evidently, the crosstalk remains low (<−20 dB) across the entire spectrum for all channels, with the overall maximum crosstalk being XT max (15,10)=−21 dB. We have also checked the crosstalk for identical waveguides separated by two superlattice periods (2 a s =10 a ), their crosstalk spectra were generally sheer noise (approximately −30 dB or lower). To further analyse the wavelength dependence of the crosstalk statistics, the transmission of all 50 crosstalk channels T ij ( j≠i ) is plotted against the direct transmission channel T ii in Fig. 4b in three wavelength bands, λ ≤1,530 nm (green), 1,530 ∼ 1,560 nm (blue) and 1,560 ∼ 1,570 nm (red). Note that for each direct transmission channel, there are 10 crosstalk channels. Evidently, the crosstalk was always lower than −20 dB in all three bands, and the crosstalk in the short wavelength band ( λ ≤1,530 nm) was even lower (<−25 dB). 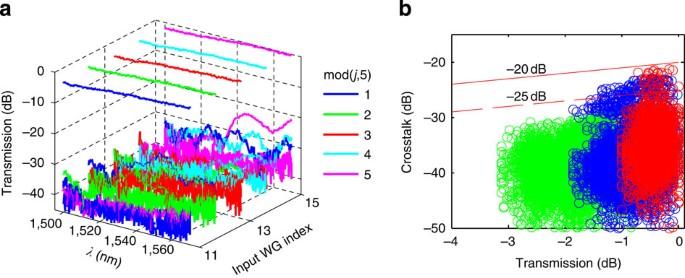Figure 4: Transmission spectra of a large-scale SC5 superlattice (made by HSQ resist) for five input waveguides in a representative supercell (Ti,j,i=11∼15,j=i−5,i−4, …i+4,i+5). a=0.78 μm,L=500 μm. The colour for each output channel is shown in the legend. (a) Spectra. To avoid cluttered view, onlyTi,i±1(λ) plus the worst are shown for eachi. (b) Scatter plot ofTi,iversusTi,jfor all 50 crosstalk spectra (j≠i), for three bands:λ≤1,530 nm (green), 1,530∼1,560 nm (blue) and 1,560∼1,570 nm (red). The lines ofTi,j−Ti,i=−20,−25 dB are delineated (to demark relative crosstalk levels). Figure 4: Transmission spectra of a large-scale SC5 superlattice (made by HSQ resist) for five input waveguides in a representative supercell ( T i,j , i =11 ∼ 15, j = i −5, i −4, … i +4, i +5). a =0.78 μm, L =500 μm. The colour for each output channel is shown in the legend. ( a ) Spectra. To avoid cluttered view, only T i,i ±1 ( λ ) plus the worst are shown for each i . ( b ) Scatter plot of T i,i versus T i,j for all 50 crosstalk spectra ( j≠i ), for three bands: λ ≤1,530 nm (green), 1,530 ∼ 1,560 nm (blue) and 1,560 ∼ 1,570 nm (red). The lines of T i,j −T i,i =−20, − 25 dB are delineated (to demark relative crosstalk levels). Full size image To assess the width control in fabrication, the waveguide widths of a SC5 superlattice fabricated by HSQ resist have been characterized by high-resolution SEM as shown in Fig. 5 . The width statistics of five waveguides in a supercell are shown in Fig. 5b . In reference to the mean width < w 1 > of the widest waveguide, the mean width differences (< w n >−< w 1 >) of the other waveguides are −60, −119, −26 and −87 nm, respectively, in good agreement with the designed values of −60, −120, −30 and −90 nm. The standard deviations of all waveguide widths are <2.7 nm. Note that the mean values of all waveguide widths had an overall shift ∼ 12 nm from the designed values. This overall shift does not change the crosstalk significantly as long as the width difference among the waveguides is retained, according to our simulation (see Supplementary Fig. 2 ). In other words, our design is robust against such an overall drift. 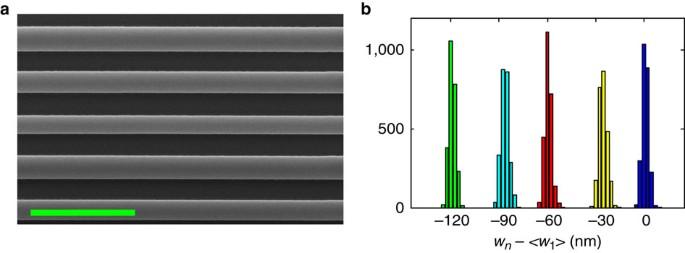Figure 5: Width statistics. (a) SEM micrograph of one supercell in a SC5 superlattice made by HSQ (scale bar, 2 μm); (b) width distribution in reference to <w1>. Figure 5: Width statistics. ( a ) SEM micrograph of one supercell in a SC5 superlattice made by HSQ (scale bar, 2 μm); ( b ) width distribution in reference to < w 1 >. Full size image The waveguide superlattice demonstrated here can potentially help to significantly improve the integration density of waveguide elements, thereby enabling higher level of integration and more advanced functionality in a given chip area and reducing the on-chip estate and cost of waveguide elements. In Si microelectronics, continual reduction of size and cost of transistors and increase of transistor density have driven the technology growth for decades (as encapsulated by Moore’s law). In photonics, increasing the density of waveguides, which are perhaps the most ubiquitous elements in integrated photonics, has been challenging due to significant crosstalk at small pitches. This work shows that pronounced increase in waveguide density can be achieved by designing sophisticated superlattices that drastically suppress crosstalk. Such high-density waveguide superlattices with fine pitches can help to significantly enhance device performance/functionality and/or reduce device area and cost. For example, in wavelength multiplexers/demultiplexers based on echelle gratings [25] , [26] , a key performance metric, the wavelength resolution between adjacent channels (Δ λ ), is proportional to the pitch of the input/output waveguide array and scales inversely with the overall device size [25] . Using a sub-micrometre-pitch waveguide superlattice at input/output can result in salient improvement of wavelength resolution, which would otherwise require a device occupying a significantly larger area. Similar use may be found in some other types of wavelength multiplexers and spectrometers. High-density waveguide superlattices can also potentially enable ultra-dense space-division multiplexing (SDM) [22] , [39] at the chip scale for optical interconnects in future high-performance computer chips, which may comprise >100 cores per chip [24] . Using large waveguide arrays with >16,000 channels for such applications was discussed (although not using the term SDM explicitly) and the large area occupied by waveguide arrays due to relatively large pitches ( ∼ 3 μm) was a major concern [24] . High-density waveguide superlattices demonstrated here can significantly reduce the area needed for SDM. This can potentially make SDM more attractive to partially substitute for or be used jointly with wavelength-division multiplexing (WDM) in some application scenarios, considering dense WDM devices are temperature sensitive and relatively complicated. As the waveguide pitch shrinks to the λ /2 mark (note a = λ /2 for λ =1,560 nm in Fig. 4 ), some technologies may advance into a new regime. For example, a phased array ideally requires emitters with λ /2 pitches to achieve maximal beam steering range. Half-wavelength pitches are routinely used in microwave-phased arrays, but have been a challenge for optical-phased arrays (OPAs) [20] , [40] , [41] . The current waveguide superlattice can be used in certain silicon-based OPA configurations [18] , [19] to deliver phase-modulated signals to an array of output waveguide-facets (or waveguide-gratings) radiating signals at λ /2 pitches, which results in λ /2-pitch optical-phased arrays. Note that the width difference has no significant impact on the OPA performance and the associated phase-shift difference can be readily compensated (see detailed discussion in Supplementary Note 4 ). Extension to two-dimensional OPA is also possible with the help of membrane transfer and stacking technology [42] . Further down-scaling of the waveguide pitch can potentially be achieved through more sophisticated superlattice structures, tighter control of the waveguide width and roughness, and even modification of individual waveguide heights. These methods can also be used to reduce crosstalk at a given pitch. For example, one may vary the waveguide widths in SC3 or SC5 structures to further reduce the crosstalk. Given w max =450 nm and w min =330 nm, one can vary w 2 in SC3 structure or individually vary w b , w c , w d in the SC5 structure to further optimize the crosstalk. Due to a large design space for all possible SC3 and SC5 superlattices, only some preliminary simulations are conducted to sample the most-promising design subspaces. Our preliminary simulations indicate that large variation (δ w >25 nm) tends to make the highest crosstalk channel of the superlattice become worse. Small variations (<10 nm for SC3 and <5 nm for SC5) may, in some cases, improve the leading crosstalk channels slightly (by 1 ∼ 2 dB). Such small improvement is close to the noise/fluctuation range of typical measurement and is not easy to experimentally differentiate. Increasing the superlattice order (for example, SC6) may reduce the inter-supercell crosstalk. But for high-order superlattice, the widths difference between waveguides in each supercell tend to decrease also. As such, intra-supercell crosstalk tends to be more sensitive to waveguide width deviation during fabrication. Currently, the crosstalk of a SC5 structure is reasonably low for a ∼ λ /2. For pitches substantially < λ /2, it might be necessary to use higher-order superlattices to combat the further rising of inter-supercell crosstalk. Simultaneously, better fabrication technology is needed to tightly control waveguide widths to minimize sensitive increase of intra-supercell crosstalk due to small waveguide width deviation. The fundamental limit of the crosstalk of a waveguide superlattice, for a given pitch a , can be considered from two aspects: physics limit and fabrication limit. Generally, the physics limit of crosstalk in a waveguide superlattice is still an open question. However, under certain assumptions, some estimate may be possible. For example, assuming that a supercell is well designed so that the worst intra-supercell crosstalk occurs between nearest neighbours (assumption 1), one can estimate the limit of overall maximum intra-supercell crosstalk by calculating the limit of maximum crosstalk of any two nearest-neighbour waveguides . Further assuming their crosstalk is not influenced by other waveguides (assumption 2), XT ( w n , w n ±1 , a ) can be computed relatively fast without knowing the surrounding waveguides; one can then use some optimization algorithm to find XT opt for all possible sets of { w n } for w min < w n < w max and a given a . To ensure assumption 1 is satisfied, it is possible to incorporate this assumption into the optimization through certain relatively loose constraints (for example, w n − w n±2 >δ 2 nm, w n − w n±3 >δ 3 nm, …), which can be developed on the basis of certain semi-analytic theory. If such constrained XT opt can be solved, one can use the experience to further tackle the problem without the two assumptions, which will be much more challenging because of the huge design space. Detailed discussion is beyond the scope of this work. The fabrication limit stems from the fact that fabrication facilities determine the roughness and width accuracy of the waveguides. Roughness influences inter-supercell crosstalk. Width accuracy determines how well a design can be implemented, particularly when the width difference is small for some high-order superlattices. These fabrication limits should be considered on the basis of the facilities available. Note that the dimension control required in the current work is well within the reach of the state-of-the-art silicon foundries [43] and, therefore, is amenable to mass production. The superlattice lengths in this work are sufficient for some applications such as wavelength (de)multiplexers [25] , spectrometers and optical-phased arrays [18] , [19] , where only a short segment of high-density waveguide array is needed at the input/output to achieve high wavelength resolution or maximal beam steering range and then the dense waveguides can be spread out through waveguide bends to connect/couple to other part of the devices/systems. In longer superlattices, our simulations show that the mean crosstalk does not change significantly and the standard deviation of crosstalk tends to increase very slowly with L (see Supplementary Fig. 4 ). Fabrication of longer superlattices can be done in mass-production-grade Si foundries, which can offer tight process control (for example, roughness control and particle contamination control) over a large area. More discussion can be found at the end of Supplementary Note 3 . Experimental results of a SC5 superlattice of different length can be found in Supplementary Fig. 6 and Supplementary Note 5 . Note that reduction of crosstalk for a pair of waveguides has been experimentally studied [44] in accordance with the well-known asymmetric directional coupler theory, but no clear route has been provided to scale the approach up to a large array. As shown in Supplementary Fig. 1 , simply replicating such an asymmetric pair of waveguides to form a SC2 superlattice will result in very poor crosstalk at sub-micrometre pitches (about −4 dB at a =0.8 μm, in contrast to <−20 dB crosstalk in a SC5 superlattice at this pitch based on the ‘interlacing-recombination’ design). Note that in many applications such as wavelength (de)multiplexers [20] , [40] , [41] , spectrometers and optical-phased arrays [25] , [26] , the number of waveguides in the input/output arrays can be fairly large. The superlattice approach can reduce crosstalk for a large number of waveguides whereas the prior approach applies only to two waveguides. Also note that plasmonic waveguides have the potential of achieving high waveguide density, but significant loss fundamentally limits their use in most practical applications. Note that waveguide bends tend to cause leakage of light. For densely packed waveguide bends (for example, a curved waveguide superlattice), leaked light can cause additional crosstalk. Generally, the leakage of light and the crosstalk increase are expected to be negligible for large bending radii; but a dense waveguide superlattice should avoid going through an abrupt bend. Further research is needed to study the relation between the crosstalk increase and the bending radius for a curved waveguide superlattice. In routing applications that have to use curved segments of waveguide array, the system-level design usually has a natural tendency—owing to bending loss concerns—to minimizing the number of bends. In such a scenario, before a dense waveguide superlattice enters a curved segment, its waveguide elements can first be spread out to a (normally used) larger pitch (for example, a >5 μm), then go through bends in this pitch with a normally used radius to achieve low crosstalk. After the curved segment, it can contract to small pitch again. As such, the crosstalk in the curved segment shall be small, comparable to that of a normal curved waveguide-array with a large pitch. The spread-out/contracting regions increase the area. As long as the curved segments are few and the total length of each waveguide is long, this area increase should be small compared with the area saving in straight segments of dense waveguide superlattice. For a multiplex/de-multiplexer based on echelle-gratings, sometimes bends are used in the routing waveguides [25] that are connected to its input/output waveguides. The wavelength-resolution improvement of a multiplex/de-multiplexer is due to the small pitch of input/output waveguides, and is not affected by the pitch of subsequent routing waveguides. Therefore, the input/output waveguide superlattice can be spread out to a large pitch (for example, a >5 μm), then connect to the routing waveguides of same pitch, and go through bends with low crosstalk. For a 30-channel echelle-grating-based de-multiplexer [25] , the extra area due to the spread-out region is estimated on the order of 0.01 mm 2 , which is small compared with the device area ∼ 0.5 mm 2 (For reference, without a superlattice of a ∼ 0.8 μm, a de-multiplexer with output waveguide pitch a ∼ 3 μm needs to increase its device area by several times to achieve same wavelength resolution). Note that here a curved waveguide-array refers to all waveguides turning ‘simultaneously’ (or concentrically) with the same starting point along the longitudinal axis. For bends in the spread-out region, the starting point of each bend can differ, so as to spatially separate the bends and reduce crosstalk (see details in the Methods). The waveguide superlattice can also stimulate new directions in scientific studies. By introducing optical nonlinearity, waveguide superlattices may provide a playground for studying a rich spectrum of phenomena in nonlinear optics, disordered systems and their interplay [27] , [45] , [46] . For example, with nonlinear self-focusing in a discrete system, we can further enhance light ‘localization’ in each ‘atom’ (waveguide), which will effectively reduce crosstalk and may enable even smaller pitches. As another example, phonon scattering of electrons in atomic crystals can be emulated by roughness-induced light scattering. Note that roughness effectively introduces a random phase dither Δ β rough , which deters coherent coupling between ‘identical’ waveguides in neighbouring supercells (see details in Supplementary Note 2 ). Hence, the results of this work suggest that the random nature of roughness/phonon may play two contrasting roles: it frustrates coherent coupling between identical atoms whereas induces incoherent scattering into non-identical atoms, resulting into two opposite localization trends. Such a complex localization behaviour in a precisely designed superlattice may shed new light on metal–insulator transition in complex crystals. Note that many scientific studies may use different characterization schemes, such as imaging the optical field of an entire lattice, rather than characterizing the crosstalk between individual waveguides. The latter is more common for optical device applications of interest here. Also note that the structures considered in this study resemble an insulator with hopping-type transport and are better described on the basis of individual waveguide modes rather than periodic Bloch modes [27] , [47] . In summary, a high-density waveguide superlattice at a half-wavelength pitch has been demonstrated with very low crosstalk. Such waveguide superlattices can significantly improve the waveguide density limit and/or the associated performance limits for a variety of Si photonic devices and systems such as wavelength multiplexer/de-mulitplexers, spectrometers, space-division multiplexing architectures and optical-phased arrays, to name a few. Waveguide superlattices can also provide a novel arrangement for exploring a host of intriguing scientific problems such as Anderson localization. Waveguide-array fabrication The waveguide superlattice structures in this work were fabricated by processes for making high-quality silicon nanophotonic structures [48] . Starting from a silicon-on-insulator wafer with a 2 μm buried oxide layer and a 260 nm top Si layer, a JEOL JBX-6300FS high-resolution e-beam lithography system was used to pattern the waveguide structures. The e-beam resists that we used were either ma-N 2405 (Micro Resist Technology) or hydrogen silsesquioxane (Dow Corning). The effects of the resist choice on sidewall roughness and light scattering are discussed in detail in Supplementary Note 2 . Then the pattern was transferred to the top silicon layer of the wafer by reactive ion etching in an Oxford Plasmalab 100 ICP etcher. Finally, a 2 μm thick silicon oxide cover was deposited by plasma-enhanced chemical vapour deposition. To facilitate measurement, the input and output ends of the waveguide superlattices were spread out to a large spacing through waveguide bends with radii ≥100 μm (radii=50 μm for the five-period superlattice to reduce the lateral pattern size), followed by a 100-μm-long taper to a 450-nm-wide access waveguide. In the spread-out region, waveguide #1 first spreads out through a commonly used S bend, waveguide #2 travels another 5 ∼ 10 μm along its axis before spreading out through an S bend, and so on. In this way, the S bends of adjacent waveguides are sufficiently separated in space, which prevents potential crosstalk increase in the bends. The propagation loss of the silicon waveguides fabricated by HSQ resist ranges from ∼ 0.6 dB mm −1 to ∼ 0.9 dB mm −1 as the width decreases from 450 nm to 330 nm. The loss difference (propagation, taper loss) between waveguides of different widths is estimated at <0.8 dB for the superlattices patterned by HSQ (actual loss had random fluctuation up to 2 dB). The propagation loss of waveguides made by ma-N is higher (about twice of those made by HSQ). For those applications requiring a short waveguide length (for example, L <500 μm for input/output waveguide arrays in WDM de-multiplexers and for output waveguides in optical-phased arrays), the loss difference of the structures fabricated by HSQ is reasonably small (<0.8 dB). For applications needing longer superlattices, two techniques can be used to address the issue of loss difference. (1) With improved fabrication in the state-of-the-art foundries, propagation loss for all waveguide widths will be reduced, and the loss difference between narrow and wide waveguides will be reduced also. (2) If necessary, power equalization between channels (for example, using a variable optical attenuator for each channel) may be applied to compensate for loss difference. Power equalization is commonly used to compensate for power difference in multi-channel systems such as WDM systems (for example, used to balance the gain (gain-flattening) between different WDM channels for Er-doped fibre amplifiers [49] ). Characterization To characterize the transmission spectra of a waveguide superlattice, light from a superluminescent LED with a spectral range of ∼ 80 nm was coupled to the TE mode of a waveguide in the superlattice via a lensed fibre. The spectra of the output light from this waveguide and other waveguides were measured by an optical spectrum analyser (OSA). Owing to mode-size mismatch between the lensed fibre (Gaussian spot size ∼ 2.5 μm) and silicon waveguides, a portion of light from the input fibre did not enter the silicon waveguides but strayed outside. A small fraction of the stray light reached the output edge of the chip and entered the output lensed fibre. The amount of stray light entering the output lensed fibre was estimated around −60 dB, in reference to the input light from the lensed fibre, in typical experiments. For long wavelengths far from the peak of the broadband source we used, the source intensity could be fairly low (for example, ∼ 10 dB down from the peak). Adding an effective attenuation of 40 ∼ 50 dB (>20 dB due to propagation and coupling loss, 20 ∼ 25 dB due to relative crosstalk), the crosstalk signal of the output waveguides at long wavelengths could diminish to a level comparable to the noise floor of the OSA. The above factors (relatively weak crosstalk signal, stray light and noise floor of the OSA) limited the lowest crosstalk that can be measured. The crosstalk reported here is measured on a waveguide-to-waveguide basis. In systems where all waveguides carry light, the overall crosstalk of a waveguide is a sum of coupled light from all other waveguides. Our simulations and experiments indicate that in a well-designed superlattice, the overall crosstalk is dominated by contributions from one or two other waveguides and contributions from all other waveguides are usually very small. For example, for the SC5 superlattice in Fig. 3e , the overall crosstalk of waveguide #7 is dominated by contributions from two waveguides, XT max (6,7)=−21.7 dB and XT max (8,7)=−25.5 dB. Contributions of all other waveguides are <−30 dB. (as discussed above, the measured crosstalk values of these channels are limited by noise floor of our setup and the actual values can be much lower). Assume all waveguides have equal input power, the overall crosstalk summed from contributions of all other waveguides will be <−20.2 dB for the worst waveguide channel. Note that optical-phased arrays often use equal power among channels [20] , [40] , [41] . In many WDM systems, the optical power values in channels are often balanced/equalized [49] . How to cite this article : Song, W. et al . High-density waveguide superlattices with low crosstalk. Nat. Commun . 6:7027 doi: 10.1038/ncomms8027 (2015).